Graphene-modified LiFePO4cathode for lithium ion battery beyond theoretical capacity The specific capacity of commercially available cathode carbon-coated lithium iron phosphate is typically 120–160 mAh g −1 , which is lower than the theoretical value 170 mAh g −1 . Here we report that the carbon-coated lithium iron phosphate, surface-modified with 2 wt% of the electrochemically exfoliated graphene layers, is able to reach 208 mAh g −1 in specific capacity. The excess capacity is attributed to the reversible reduction–oxidation reaction between the lithium ions of the electrolyte and the exfoliated graphene flakes, where the graphene flakes exhibit a capacity higher than 2,000 mAh g −1 . The highly conductive graphene flakes wrapping around carbon-coated lithium iron phosphate also assist the electron migration during the charge/discharge processes, diminishing the irreversible capacity at the first cycle and leading to ~100% coulombic efficiency without fading at various C-rates. Such a simple and scalable approach may also be applied to other cathode systems, boosting up the capacity for various Li batteries. The serious climate change concern coupled with high fuel prices are driving the research and investment in the development of sustainable energies, such as solar energy, wind energy, hydroelectricity, wave power and geothermal energy. The sustainable energy, after its generation, needs to be efficiently stored for future use in devices as well as vehicles. The development in energy-storage devices with high capacity and power has progressed at an unprecedented high speed over last decade. Li ion battery is one of the most promising solutions for these storage systems because of its outstanding electrochemical performance and high capacity. To meet such a strong demand in higher-capacity storage, the rate capability and energy density of Li + ion battery must be improved, which urges the discovery of a novel composite cathode or anode. Lithium iron phosphate (LiFePO 4 or LFP), one of the very popular commercial cathode materials for Li battery, exhibits several advantageous features for the energy storage such as low cost, environmental capability, relatively large capacity and intrinsic stability. Not unique to the LFP, all cathode materials exhibit their theoretical value in charge capacity, which is limited by intrinsic property of the material. Structural defects or other factors that may retard the Li + diffusion further lower the actual capacity of the cathode. Current strategies to enhance the electrochemical performance of LFP include carbon coating on LFP (cLFP) [1] , [2] , [3] , [4] , [5] , [6] , metal doping [7] , [8] , [9] , and LFP particle size reduction [10] , [11] , [12] , [13] , [14] , [15] . The carbon coating process has been massively used in industry because the conductive carbon layer increases the electron migration rate during the charge/discharge processes. Metal doping is able to expand the Li + diffusion channel and increase the output voltage of LFP-based Li ion battery. The reduction of LFP particle size results in the shortening of the Li + diffusion path; however, the disadvantage is that the high surface area requires higher loading amount of binders to glue these small LFP particles together, where the inclusion of binders further decreases the capacity. Hence, the nano-sized materials are still not applicable to practical Li ion batteries. Recently, graphene has become the spotlight in lithium ion battery research because it owns several desirable features, including high surface area and excellent electronic conductivity, for improving the electrochemical performance of LFP. The most popular approach to synthesize graphene is to reduce the chemically exfoliated graphene oxide (GO) obtained by Hummer’s method, owing to that the method is potentially scalable. Several reports have demonstrated some enhancement in rate capacity using the reduced GO (rGO)/LFP composite material as the cathode, where the cathode was prepared by pyrolyzing the GO or rGO together with either LFP precursors or LFP particles [16] , [17] , [18] , [19] . The capacity increase was attributed to that the rGO sheets helped to enhance the electron transport rate in cathodes. The specific capacity of the rGO-modified LFP cathodes in these reports ranged from 146 to 165 mAh g −1 . Here we report that the incorporation of few-layer graphene obtained by another scalable method electrochemical exfoliation [20] is able to deliver a capacity of 208 mAh g −1 , which is beyond the theoretical capacity of LFP 170 mAh g −1 . The energy density is up to 686 Wh kg −1 , much higher than the typical 500 Wh kg −1 of LFP. The excess capacity is attributed to the ultrahigh capacity (>2,000 mAh g −1 ) of the electrochemically exfoliated graphene (EG) flakes. The cyclic voltammetric measurement for the half cells with EG flakes as the only active material reveals the reversible redox reaction that contributes to the Li + ion storage capacity. The capacity enhancement effect is obvious such that only a very low weight percentage of graphene (<2 wt%) is required, and the low loading percentage avoids the unwanted voltage polarization effect that can been seen after introducing higher graphene percentage in cathodes. Meanwhile, the superior quality of the electrochemically EG, with a relatively higher carrier mobility compared with available rGO, greatly enhances the electron transfer during the charging and discharging processes. It is noteworthy that only ~0.8 and 2 wt% of graphene is needed to achieve the capacity 187 and 208 mAh g −1 , respectively, without causing unfavourable voltage polarization. Electrochemically exfoliated graphene Large quantity of EG thin flakes were prepared using an electrochemical exfoliation method previously reported by us [20] . In brief, a graphite rod was used as the source that can be exfoliated to produce graphene layers during the electro-oxidation process. A platinum wire was used as a grounded electrode, and the electrolyte solution has been optimized (SO 4 2− at pH ~12 as described in Methods) to serve efficient exfoliation but without severely degrading the graphene layers. Once a sufficiently high bias (10 V) was applied to the graphite rod, it was quickly dissociated into small flakes spreading on the solution surfaces. These EG flakes were collected by filtration and then re-dispersed in dimethylformamide (DMF). The as-dispersed graphene solution in DMF was further centrifuged to remove the unwanted side products, thick graphite particles. We have optimized the centrifugation condition to obtain the graphene layers with a narrowed distribution in thickness. 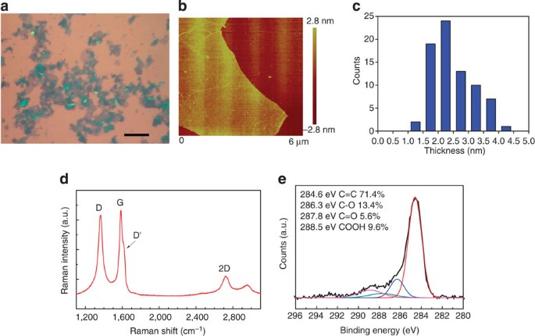Figure 1: Characterization of electrochemically exfoliated graphene flakes. (a) Optical micrograph for the graphene ensemble. Scale bar, 15 μm. (b) AFM image of a selected graphene flake. (c) Statistical measurement results of AFM thickness for randomly selected 76 flakes, where the thickness ranges from 1.5 to 4.2 nm (d) Typical Raman spectrum (excited by a 473 nm laser) and (e) C1s binding energy profile measured by X-ray photoemission spectroscopy for the obtained few-layer graphene ensemble. Figure 1a displays the typical optical micrograph, and Supplementary Fig. S1 shows the scanning electron microscope (SEM) image for the graphene flake ensemble we used in this study, where the lateral size of the flakes ranges from a few to several tens of μm. Figure 1b displays the atomic force microscope (AFM) image of a selected graphene flake. Figure 1c shows the statistical measurement results of AFM thickness for randomly selected 76 flakes from the ensemble, where the thickness ranges from 1.5 to 4.2 nm (average 2.5 nm). Figure 1d shows the typical Raman spectrum and the binding energy profile measured by X-ray photoemission spectroscopy, respectively. The observation of Raman D and D′ bands, as well as the X-ray photoemission spectroscopy C1s binding energies at 286.4 eV (C-OH), 287.8 eV (C=O) and 288.9 eV (O=C-OH), suggests that some oxygen-containing functional groups are present, where the atomic percentages of various carbons derived from the fitted peak areas are indicated in Fig. 1e . However, the existence of a sharp two-dimensional band (~2,700 cm −1 ) indicates that the few-layer EG flakes are still with reasonably good graphitic structures, where their conductivity is superior to commonly used GO or rGO sheets [20] . Figure 1: Characterization of electrochemically exfoliated graphene flakes. ( a ) Optical micrograph for the graphene ensemble. Scale bar, 15 μm. ( b ) AFM image of a selected graphene flake. ( c ) Statistical measurement results of AFM thickness for randomly selected 76 flakes, where the thickness ranges from 1.5 to 4.2 nm ( d ) Typical Raman spectrum (excited by a 473 nm laser) and ( e ) C1s binding energy profile measured by X-ray photoemission spectroscopy for the obtained few-layer graphene ensemble. Full size image Morphology of the graphene-coated LiFePO 4 In the study, we used commercially available LiFePO 4 powders (particle diameter ~300 nm), and these as-received particles were coated with a thin amorphous carbon layer (cLFP). To achieve homogenous coating of few-layer graphene flakes on the surface of cLFP, the DMF solution of EG flakes (concentration ~250 p.p.m.) was dropwise added to cLFP powders with gentle stirring at 180 °C. The EG flakes spread in the mixture with the aid of DMF solvent and wrapped the surfaces of cLFP particles through van der Waals interaction. Meanwhile, the DMF solvent gradually evaporated at the mixing temperature. The SEM image in Fig. 2a illustrates that the EG flakes nicely cover the cLFP particles after added to cLFP. 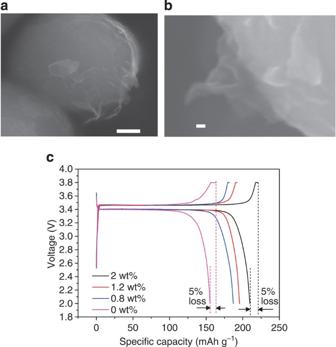Figure 2: Specific capacity of the graphene-coated LiFePO4. (a,b) SEM images of the carbon-coated LiFePO4particles wrapped by electrochemically EG sheets. Scale bar, 100 nm and 10 nm (inaandb, respectively). (c) The voltage profiles for the first cycle charging and discharging (with a rate of 0.1 C) of the carbon-coated LiFePO4cathodes with various graphene-loading percentages (0, 0.8, 1.2 and 2 wt%). Figure 2b shows the magnified SEM image, where the wrinkles of the graphene layers are clearly observed. Coin-sized half-cells with various cathode compositions, for example, cLFP materials with and without the addition of few-layer EG, were assembled using a lithium foil as the anode. Figure 2: Specific capacity of the graphene-coated LiFePO 4 . ( a , b ) SEM images of the carbon-coated LiFePO 4 particles wrapped by electrochemically EG sheets. Scale bar, 100 nm and 10 nm (in a and b , respectively). ( c ) The voltage profiles for the first cycle charging and discharging (with a rate of 0.1 C) of the carbon-coated LiFePO 4 cathodes with various graphene-loading percentages (0, 0.8, 1.2 and 2 wt%). Full size image Specific capacity of the graphene-coated LiFePO 4 The charging/discharging voltage profile for the cell using the cathode loaded with a very low EG percentage of 0.13 wt% does not show much difference compared with that using the cathode loaded with only cLFP ( Supplementary Fig. S2 ). Figure 2c shows that the voltage profiles of the first cycle with 0.1 C as the charging and discharging rate for the cathodes with higher EG loading percentages become drastically different from that without EG. The EG-wrapped cLFP cathodes provide the capacity from 187 to 208 mAh g −1 , depending on the weight percentage of EG (from 0.8 to 2 wt%). These values are higher than the reported values of 120–160 mAh g −1 for commercially available or synthetic LFP materials in research laboratories [16] , [17] , [21] , [22] . Surprisingly, these values are even in excess of the theoretical value of 170 mAh g −1 for LFP. Supplementary Fig. S3 plots the specific discharge capacity value as a function of the percentage of EG based on the results of Fig. 2c , where the discharge capacity of the EG, layers in the 2 wt% sample is estimated to be as high as 2,720 mAh g −1 . It has been well established that the major LFP capacity is attributed to the Li + insertion to and extraction from the LFP particles (chemical equation: LiFePO 4 =FePO 4 +Li + +e − ). Two major limiting processes have been reported to explain why some lithium ions cannot be fully extracted from the ordered-olivine structure which in turn causes some capacity loss. (i) Limited lithium ion phase-boundary diffusion: the one-dimensional channels in LFP impose structural constraint, where the Li + diffusion can be interrupted by ionic disorder, foreign phases or stacking faults. Interruption of Li + diffusion impedes the motion of a LiFePO 4 /FePO 4 phase boundary that removes portions of the cathode from accessing to a reversible Li + intercalation [23] . (ii) Low electron conductivity: during the charging and discharging processes, the charges must be kept in balance with the insertion/extraction of Li + via electron transfer. If electrons are not able to transfer rapidly, the electron mobility will limit the Li + insertion/extraction and cause a deteriorated electrochemical property. To resolve these issues, many attempts have been made to expand the one-dimensional channels of the olivine structure for smooth Li + diffusion, such as the doping with impurities, metals or metal oxides [24] , [25] , [26] . Alternatively, significant effort has been devoted to coating the LFP surfaces with electrically conductive materials, such as amorphous carbon and conducting polymers to enhance the electrical conductivity of LFP surfaces [27] , [28] , [29] , [30] , [31] , [32] . Recent studies have adopted rGO or GO to cover the LFP surfaces [16] , [17] , [18] , [19] . However, studies so far have only shown certain improvements in the rate capability but no report has exceeded the theoretical limit of the capacity. Therefore, enhanced capacity over the theoretical value by adding EG layers must be associated with the unique features of EG layers. 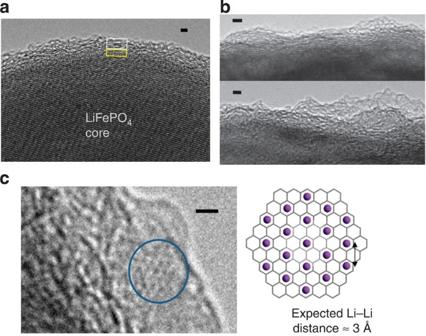Figure 3: TEM images. High-resolution TEM images of the carbon-coated LiFePO4cathode materials with 0.8 wt% of graphene (a) after charging (Li+extraction), where the yellow square indicates the amorphous carbon coating and the white square is the added graphene layers. Scale bar, 1 nm. (b) After discharging (Li+insertion), the graphene layer-to-layer distance expands and becomes disordered in stacking. Scale bar, 1 nm. (c) The in-plane view of the graphitic layers at the edge of the carbon-coated LiFePO4particle, which shows a possible indication of hexagonal lattice that is typically formed by Li+ion intercalated graphite. Scale bar, 0.7 nm. Figure 3a shows the high-resolution transmission electron microscopy (HRTEM) image for the cLFP cathode materials with 0.8 wt% EG after charging (Li + extraction from the cathode), where the cathode material was obtained by cleaving the Li-battery half-cell immediately after the charging procedure. HRTEM reveals that the initial amorphous carbon coating on cLFP particles is around 1-nm thick, and the thickness of EG on top of the amorphous carbon is 1.5–2 nm (only few layers) for the selected site. Most of the graphene layers seem to stack around the surface of the cLFP particle. Figure 3b displays the HRTEM images after the cathode material is discharged (Li + insertion to the cathode). It is observed that graphene layers become very disordered, with many layers oriented randomly with respect to the surface of the cLFP particle. Furthermore, statistical measurements of distances between graphene layers show an increase for the average interlayer distance from 0.32 nm for the charged cathode to 0.38 nm for the discharged one ( Supplementary Fig. S4 shows the TEM analysis of graphene layer-to-layer distances for over 12 sites). These observations indicate that Li + ions come into the few-layer EG after discharging, resulting in the expansion of interlayer distance. Note that it is not easy to visualize individual Li + ions in HRTEM; however, the occasionally found in-plane view of the graphitic layers at the edge of the cLFP particle as shown in Fig. 3c shows a hexagonal periodicity that is typical for the two-dimensional lattice of Li + ions intercalated in graphite, providing an alternative proof for Li + ions insertion to EG. Figure 3: TEM images. High-resolution TEM images of the carbon-coated LiFePO 4 cathode materials with 0.8 wt% of graphene ( a ) after charging (Li + extraction), where the yellow square indicates the amorphous carbon coating and the white square is the added graphene layers. Scale bar, 1 nm. ( b ) After discharging (Li + insertion), the graphene layer-to-layer distance expands and becomes disordered in stacking. Scale bar, 1 nm. ( c ) The in-plane view of the graphitic layers at the edge of the carbon-coated LiFePO 4 particle, which shows a possible indication of hexagonal lattice that is typically formed by Li + ion intercalated graphite. Scale bar, 0.7 nm. Full size image In fact, the intercalation of Li + ions into graphite is typically seen in the electrochemical process occurring in a graphite anode; nevertheless, the theoretical capacity is ~372 mAh g −1 and the reversible intercalation of lithium in graphite occurs at only ~0.1 V that is far to the 3.4 V. Highly disordered graphene nanosheets have been shown to exhibit a higher reversible Li + ion storage capacity up to 1,100 mAh g −1 . However, the charge/discharge profiles should be with a large voltage hysteresis and without distinct potential plateaus [33] . These indicate that there should exist another Li + ion storage mechanism for the observed high capacity from EG. To reveal the possible origin of the excess capacity, we deposit EG flakes on inactive silica particles (diameter ~5–10 μm) as cathode materials and make coin-sized cells following the same method used for EG/cLFP. This allows us to directly measure the capacity of EG flakes. The second cycle voltage profiles of the cathodes made by 0 and 1.8 wt% EG on silica particles (EG/silica) are shown in Supplementary Fig. S5 . It is observed that silica particles exhibit a small reversible capacity, whereas EG flakes demonstrate a significantly large reversible capacity. 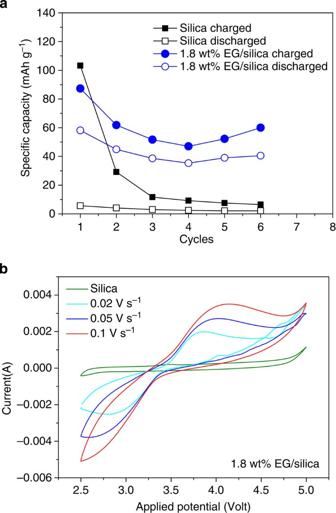Figure 4: The electrochemical characteristics. (a) The cycling properties for the coin cells with the cathodes made by 0 and 1.8 wt% graphene flakes on silica particles. Charge/discharge rate: 23 mA g−1. (b) The cyclic voltammetry characteristics for these two cells. The curve for silica was collected at a rate of 0.02 V s−1. Figure 4a compares their cycling properties at a fixed charge/discharge current density 23 mA g −1 , corresponding to 0.5 and 7.5 C of rate capabilities for the cathodes with 1.8 and 0 wt% EG, respectively. The rate capability of 1.8 wt% EG/silica remains after six cycles; however, the rate capability of pure silica fades after a few cycles. This result indicates that EG flakes incorporated with the cathode materials is able to enhance the capability of Li + ion storage from EG, and this storage mechanism is reversible. Based on Fig. 4a , the charge (discharge) capacity for the 1.8 wt% EG/silica at the sixth cycle is 53.5 (38.3) mAh g −1 higher than that for pure silica, where the specific charge (discharge) capacity of EG is estimated to be ~2970 (2,120) mAh g −1 , consistent with the high capacity obtained in Supplementary Fig. S3 . As the preparation of EG involves electrochemical reactions in a solution, it is very likely some redox active sites or defects are activated and remained on EG, where the sharp Raman D-band in Fig. 1 is perhaps the good indication for the presence of defects. Figure 4b shows the cyclic voltammetry characteristics for these two coil cells at various scan rates. No redox peak for silica particles is observed because the potential of the Li + ion intercalation and extraction of silica is between 0.2 and 0.5 V. The slow scan rate 0.02 V s −1 reveals an oxidation peak at 3.5–4.5 V and a reduction peak at 2.5–3.5 V for the sample with EG, clearly demonstrating the presence of a reversible redox reaction that can contribute to Li + ion storage capacity. Some Li + ions may be stored reversibly between graphene planes, but the redox-based reversible storage should predominate, where the defects at edge sites or basal planes (vacancies and so on) of the EG may be involved. However, it is noteworthy that special care should to taken to avoid the re-stacking when applying EG flakes to electrode materials because they tend to easily agglomerate to increase the polarization and decrease their surface areas. We have deposited EG flakes onto a flat surface to form a thick film; however, the measured specific capacity for the stacked EG flakes is only ~350 mAh g −1 , much lower than the value obtained from EG/silica cathodes. Figure 4: The electrochemical characteristics. ( a ) The cycling properties for the coin cells with the cathodes made by 0 and 1.8 wt% graphene flakes on silica particles. Charge/discharge rate: 23 mA g −1 . ( b ) The cyclic voltammetry characteristics for these two cells. The curve for silica was collected at a rate of 0.02 V s −1 . Full size image Another significant change after EG addition to cLFP is the reduction in the first cycle loss of capacity. Figure 2c shows that the irreversible capacity of EG/cLFP-based lithium battery is vanished for the cathodes loaded with 0.8 and 1.2 wt% of EG, respectively. The outstanding cycling performance is attributed to the highly conductive few-layers graphene homogenously distributed around cLFP particles, which serve as a fast path for electron migration during the charge/discharge processes [18] . It is known that electron transfer in sp 2 carbon is more effective than in sp 3 amorphous carbon [34] , [35] . The electrons are capable of spreading to the entire surface of the EG/cLPF particles through the EG sheets during charge/discharge, improving the kinetics and reversibility of the lithium insertion/extraction cycles. However, the irreversible capacity increases to 5% when EG percentage is increased to 2 wt%. The irreversible capacity is also ~5% for the cell based on cLFP cathodes without EG. Yang et al . [36] have shown that the first cycle loss percentage increases with the carbon content because lengthened Li + diffusion path caused by the overall increase in carbon content increase may hinder the diffusion. It is noteworthy that the voltage plateau for the EG/cLFP cathode-based coin cell still remains at 3.4 V, which indicates that the homogenous coating of EG does not cause the unwanted polarization effect, which is advantageous for the Li + battery. However, if the EG coating around cLFP particles is not uniform, that is, EG layers stack together, it would be reflected in additional voltage polarization. If the graphene flakes are too thick, they would behave like graphite particles that would cause the unwanted voltage polarization [37] . Such an electrochemical behaviour is typically known as for graphite particles. Supplementary Fig. S6 shows the voltage profile for the cell with the cLFP cathode loaded with 2 wt% EG but prepared with rough mixing (EG solution was not added in a dropwise manner), where the obvious voltage polarization is observed. As graphene layers tend to stack to form thicker aggregates, the structure is closer to graphite, due to the strong π−π stacking interaction. The cycle life is also increased because of the few-layer graphene coating, where the electrons can be fast transferred on the surface of cLFP to withstand the high discharging rate. For 0.8 wt% EG-wrapped cLFP, the cycle life is substantially improved at higher discharging rate, 2.5 C, comparing with commercial cLFP and lower weight percent of EG-wrapped cLFP as shown in Fig. 5a . 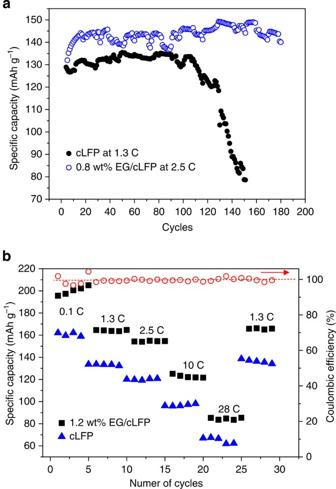Figure 5: The cycle life test for the battery. (a)The cycle life test for the Li+ion battery cells based on the carbon-coated LiFePO4cathodes added with 0 and 0.8 wt% of graphene. (b) The discharge rate capability and Coulombic efficiency at different charge/discharge rates for the Li+ion battery cells based on the cathodes added with 0 and 1.2 wt% of graphene. Figure 5b shows the discharge rate capability and coulombic efficiency at different charge/discharge rates for the lithium ion battery cells based on the cathode added with 1.2 wt% of EG. The discharge capacity performance for the reference cell based on cLFP without EG is also shown for comparison. As expected, when the discharge rate is increased, both cathodes cannot sustain a high discharging current (fast Li + intercalation) and thus the capacity fades very quickly. However, the cell loaded with EG can deliver >23% higher capacity at lower rates 0.1–1.3C and >26% higher capacity at higher C-rates 2.5–28C, consistently demonstrating the advantages of adding EG. In particular, the composite cathode material, EG/cLFP, can deliver a capacity ~125 mAh g −1 at a high discharging rate 10 C, which is around 26% better than the 98 mAh g −1 obtained from cLFP only. The Coulombic efficiency of EG/cLFP still maintains at 98–100% for various C-rates. Figure 5: The cycle life test for the battery. (a) The cycle life test for the Li + ion battery cells based on the carbon-coated LiFePO 4 cathodes added with 0 and 0.8 wt% of graphene. ( b ) The discharge rate capability and Coulombic efficiency at different charge/discharge rates for the Li + ion battery cells based on the cathodes added with 0 and 1.2 wt% of graphene. Full size image In summary, the electrochemically exfoliated few-layer graphene sheets have been applied to wrap the commercially available cathode material cLFP. The incorporation of low weight percent (2 wt%) of graphene in cLFP is able to deliver a capacity of 208 mAh g −1 , which is beyond the theoretical 170 mAh g −1 without causing obvious voltage polarization. The energy density is up to 686 Wh kg −1 , higher than the typical value 500 Wh kg −1 for cLFP. The extra capacity is mainly attributed to the reversible redox reaction between the lithium ions of the electrolyte and the EG flakes. The addition of high-capacity materials to improve the capacity of an existing cathode material, like two capacitors connected in parallel, has been proved to be successful. The wide range of the redox potential of the EG flakes is also likely applicable to other cathode materials for Li battery, and this study may stimulate extensive research into fundamentals of this process and advance industrial applications. Synthesis of electrochemically EG The preparation of electrochemically exfoliated few-layer graphene was based on the method developed in our previous report [20] as briefly described below. Natural graphite flake or graphite powders compressed as a rod was used as the graphene source as well as the working electrode. A Pt wire was chosen as a grounded electrode. An aqueous solution containing SO 4 2− (2.4 g of 98% H 2 SO 4 in 100 ml of deionized water, and added with 11 ml of 30% KOH solution to make its pH value around 12) was used as an electrolyte. The static bias of +2.5 V was first applied to the working electrode for 5–10 min, followed by ramping the bias to +10 V for graphene exfoliation. The initial low bias helps to wet the sample and likely causes gentle intercalation of SO 4 2− ions to the grain boundaries of graphite [38] , [39] . Before applying a high bias of +10 V, the graphite working electrode still remained as a single piece. Once the high bias was applied, the graphite was quickly dissociated into thin sheets and spread in the solution surface. These EG sheets and related products were collected by filtration and then re-dispersed in DMF. We note that the electrochemical exfoliation of graphene is very efficient as the whole exfoliation process can be finished in a few minutes but it generally produces thin sheets with large amounts of defects because of the fact that the H 2 SO 4 itself also results in strong oxidation of graphite. Switching the applied voltage between +10 and −10 V during the exfoliation helps to reduce the oxidation of EG layers. The large-scale synthesis and purifications of the electrochemically EG flakes used in this study were assisted and performed in Nitronix Nanotechnology Corp. (Taiwan). Synthesis of EG-wrapped LFP The electrochemically EG sheets dispersed in a DMF solution (250 p.p.m.) were dropwise added to the commercially available LiFePO 4 powders (diameter ~300 nm; from Tatung fine chemicals Co.) with gentle stirring at 180 °C. It is noted that the commercially available LFP particles were normally coated with an amorphous carbon layer; hence, we name it as cLFP. The van der Waals forces between graphene sheets and cLFP particles drive the formation of cLFP particles wrapped with graphene layers on their surfaces, as shown in Fig. 2 . The good wrappability provides good protection for cLFP particles against the volume expansion or agglomeration. The EG-wrapped cLFP was used as the active material for the electrochemical test. Electrochemical test For the preparation of the lithium ion battery cathodes, 10 wt% Super P was first mixed with 10 wt% polyvinylidene difluoride in N -methyl-2-pyrrolidone followed by the addition of 80 wt% of the active material EG/cLFP, and all were mixed with stainless steel balls for ball-milling at 400 r.p.m. The resultant slurry, pasted on an Al foil, was dried at 110 °C for 4 h. The coin cells (2032) then were assembled in an argon-filled glove box using a lithium foil as the anode, Celgard 2600 as the separator and 1 M LiPF 6 dissolved in ethyl methyl carbonate, dimethyl carbonate and vinylene carbonate with a volume ratio of 1:1:1 as the electrolyte. Cells were tested at ambient temperature. The testing voltage in the constant current mode was in a range of 2.0–3.8 V, and the cells were charged in the constant voltage mode at 3.8 V until the current reached 0.05 C. Characterizations The AFM images were performed in a Veeco Dimension-Icon system. Raman spectra were collected in a confocal Raman system (from NT-MDT company). The wavelength of laser is 473 nm (2.63 eV), and the spot size of the laser beam is ~0.5 ìm and the spectral resolution is 3 cm −1 (obtained with a 600 grooves per mm grating). The Si peak at 520 cm −1 was used as a reference for wave number calibration. For TEM, the cathode material was rinsed by ethanol and dried in the glove box. The EG/cLFP was scratched off from the Al foil and then sonicated in ethanol. The EG/cLFP in ethanol solution was dropped on a copper grid for TEM observation. HRTEM imaging was performed on JEOL 2100F FEG-TEM operated at 100 kV. How to cite this article: Lung-Hao Hu. et al . Graphene-modified LiFePO 4 cathode for lithium ion battery beyond theoretical capacity. Nat. Commun. 4:1687 doi:10.1038/ncomms2705 (2013).